Multifunctional nanoagents for ultrasensitive imaging and photoactive killing of Gram-negative and Gram-positive bacteria Simultaneous imaging and treatment of infections remains a major challenge, with most current approaches being effective against only one specific group of bacteria or not being useful for diagnosis. Here we develop multifunctional nanoagents that can potentially be used for imaging and treatment of infections caused by diverse bacterial pathogens. The nanoagents are made of fluorescent silicon nanoparticles (SiNPs) functionalized with a glucose polymer (e.g., poly[4-O-(α-D-glucopyranosyl)-D-glucopyranose]) and loaded with chlorin e6 (Ce6). They are rapidly internalized into Gram-negative and Gram-positive bacteria by a mechanism dependent on an ATP-binding cassette (ABC) transporter pathway. The nanoagents can be used for imaging bacteria by tracking the green fluorescence of SiNPs and the red fluorescence of Ce6, allowing in vivo detection of as few as 10 5 colony-forming units. The nanoagents exhibit in vivo photodynamic antibacterial efficiencies of 98% against Staphylococcus aureus and 96% against Pseudomonas aeruginosa under 660 nm irradiation. The World Health Organization (WHO) released its first Essential Diagnostics List (EDL) in 2018, highlighting the fundamental role of rapid, sensitive, specific, and reasonably priced diagnostics for effective treatments of infectious diseases caused by viruses, parasites, and bacteria [1] . Notwithstanding, it is striking that more than 300 million individuals are still killed by sepsis, endocarditis, and other pathogen-related diseases per year [2] , [3] , [4] . Currently, a promising cure strategy is to diagnose pathogen in vivo with high specificity and sensitivity and effectively eliminate them at an early stage [5] , [6] , [7] , [8] . Although there are numerous established methods developed for detection of bacteria, such as bacterial culture, biochemistry identification, immunoassays, polymerase chain reaction (PCR), sequencing and so forth, they generally require complex and time-consuming procedures (e.g., several hours to days for bacterial culture, bacterial metabolites extraction, and bacterial discrimination) to analyze results [9] , [10] . As a consequence, even though diagnosis is able to be confirmed via these approaches, the golden time for treatment is possibly missed because bacterial infections may already have caused serious anatomical tissue damage or become systemic [11] , [12] . Even in an ideal clinical environment, the physicians would usually perform the broad-spectrum and non-specific anti-bacteria treatment before diagnosis. Fluorescence imaging has been recently considered as a simple, rapid and sensitive method for bacteria detection [13] , [14] , [15] , [16] , [17] . Of note, extensive efforts have been devoted for developing illuminant nanomaterials-based theranostic agents against microorganisms, which are capable of not only diagnosis of bacterial infections but also curing bacterial infections by virtue of delivering therapeutic agents to the site of interest [14] , [18] , [19] . However, there are three major barriers limiting their widespread applications: (1) most nanoagents feature poor specificity for bacteria over mammalian cells, resulting in difficulty for distinguishing bacterial infections from other inflammation symptoms [20] , [21] , [22] , [23] ; (2) most reported nanoagents could basically determine only one specific group of bacteria (i.e., Gram-negative or Gram-positive bacteria), while clinical bacterial infections (e.g., sepsis, skin burn infection, unsterilized device infection, and so on) are generally caused by both Gram-negative and Gram-positive pathogenic bacteria [11] , [24] , [25] ; (3) currently existing nanoagents usually possess a single emission under a single excitation, their single-emission signals are therefore easily influenced by fluctuation of local probe concentration, leading to difficulty in the accurate and reliable bacterial detection [5] , [14] . As previously reported, silicon nanoparticles (SiNPs) feature benign biocompatibility, bright fluorescence coupled with strong photostability (e.g., SiNPs could preserve strong fluorescence under continuous 180-min UV irradiation) and adjustable drug-loading capacity (e.g., doxorubicin (DOX) loading content onto SiNPs can be up to 21.34%) [26] , [27] . It is noteworthy that ultrasmall SiNPs (<10 nm) recently have been approved by the Food and Drug Administration (FDA) of USA for the first-in-human clinical trial [28] , [29] , [30] . In addition, glucose polymer (GP) as the major microbial carbon source is selectively and robustly internalized into bacterial cells through GP-mediated ATP-binding cassette (ABC) transporter on the bacterial cell membrane at a high uptake rate (e.g., K m of ~130 μm) [31] , [32] , [33] , [34] , [35] , [36] , [37] , [38] , [39] , [40] . For instance, the GP-mediated ABC transporter in E. coli is comprised of five subunits: LamB, MalE, MalF, MalG, and MalK, in which MalE is responsible for recognition of linearly α (1–4)-glucosidically linked glucose polymer (e.g., amylose, starch, maltodextrin, etc.) [36] . On the contrary, GP hardly enter into mammalian cells due to the absence of GP-mediated ABC transporter on the cell membrane of mammalian cell [36] , [37] . Furthermore, chlorin e6 (Ce6), serving as another type of imaging agent, is able to provide stable red fluorescence signals as well as a photosensitizer, which can generate singlet oxygen under 660-nm illumination to kill bacterial cells [41] , [42] , [43] . Here we present multifunctional nanoagents that can be used for imaging and treatment of bacterial infections. The nanoagents (GP-Ce6-SiNPs) are made of fluorescent SiNPs functionalized with a GP and loaded with Ce6, and are taken up by bacteria via ABC transporters. By virtue of this merit, as few as 10 5 colony-forming units (CFUs) of bacteria can be imaged in vivo. Moreover, the antibacterial efficiency of the developed nanoagents is up to ca. 98% against S. aureus and ca. 96% against P. aeruginosa under 40-min exposure with a relative low power laser (660 nm, 12 mW cm −2 ). Fabrication of GP-Ce6-SiNPs As schematically illustrated in Fig. 1a , the GP-Ce6-SiNPs are composed of three ingredients; those are SiNPs, GP, and Ce6. In this system, fluorescent SiNPs covered with amine groups are synthesized through our previously reported protocol [44] . GP (e.g., poly[4-O-(α-D-glucopyranosyl)-D-glucopyranose]) as the targeted ligand is conjugated with SiNPs through the classic Schiff base reaction, in which the aldehyde groups of GP react with amino groups on SiNPs surface to form Schiff base and then reduced by NaBH 4 to form stable structure. Thereafter, Ce6 molecules are loaded onto SiNPs through electrostatic adsorption, thus yielding the theranostic nanoagents of GP-Ce6-SiNPs ready for photodynamic treatment of bacteria. Fig. 1 Design of multifunctional nanoagents for detection and photodynamic treatment of bacterial infections. a Synthetic route of nanoagents of GP-Ce6-SiNPs. GP-Ce6-SiNPs are composed of SiNPs conjugated to GP and loaded with Ce6 molecules. b Imaging and treatment of Gram-negative and Gram-positive bacterial infections by GP-Ce6-SiNPs. GP-Ce6-SiNPs are robustly internalized by ABC transporters, which are only present in bacterial cells while not present in mammalian cells. Under 405-nm excitation, GP-Ce6-SiNPs exhibit two typical emission maxima peaks at 520 nm (assigned to SiNPs) and 670 nm (assigned to Ce6). Under 660-nm irradiation, ROS of 1 O 2 is produced from Ce6, triggering PDT against bacteria. 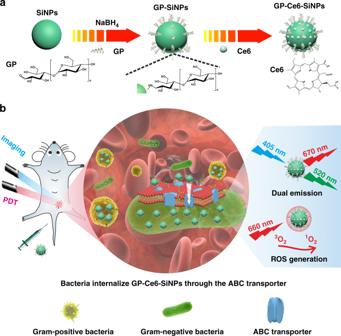Fig. 1 Design of multifunctional nanoagents for detection and photodynamic treatment of bacterial infections.aSynthetic route of nanoagents of GP-Ce6-SiNPs. GP-Ce6-SiNPs are composed of SiNPs conjugated to GP and loaded with Ce6 molecules.bImaging and treatment of Gram-negative and Gram-positive bacterial infections by GP-Ce6-SiNPs. GP-Ce6-SiNPs are robustly internalized by ABC transporters, which are only present in bacterial cells while not present in mammalian cells. Under 405-nm excitation, GP-Ce6-SiNPs exhibit two typical emission maxima peaks at 520 nm (assigned to SiNPs) and 670 nm (assigned to Ce6). Under 660-nm irradiation, ROS of1O2is produced from Ce6, triggering PDT against bacteria. The cartoons are created by Dr. Houyu Wang The cartoons are created by Dr. Houyu Wang Full size image Figure 1b illustrates the mechanism of GP-Ce6-SiNPs for the detection and photodynamic treatment of Gram-negative and Gram-positive pathogens in vivo. The mice infected by both Gram-negative and Gram-positive bacteria are injected with the GP-Ce6-SiNPs through tail vein. GP-Ce6-SiNPs can be internalized into both Gram-negative and Gram-positive bacteria through bacteria-specific ABC transporter pathway, manifesting green fluorescence of SiNPs (maximum emission wavelength at 520 nm) and red fluorescence of Ce6 (maximum emission wavelength at 670 nm) under 405-nm excitation. On the other hand, when the infected tissues are exposed to 660-nm irradiation, PDT against bacterial cells is triggered, thus producing reactive oxygen species (ROS) of singlet oxygen ( 1 O 2 ) from Ce6 based on the photoenergy transferring from Ce6 to surrounding oxygen molecules [41] , [42] , [43] . Characterization of GP-Ce6-SiNPs A series of experiments are performed to characterize the as-prepared GP-Ce6-SiNPs. 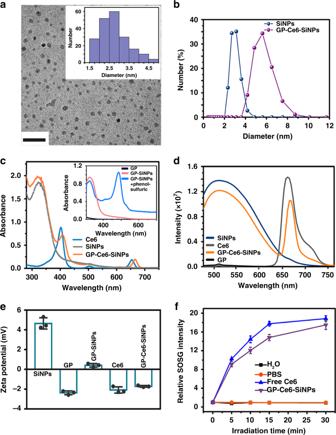Fig. 2 Characterization of GP-Ce6-SiNPs.aTEM image and corresponding size distribution (inset) of GP-Ce6-SiNPs. Scale bar: 20 nm.bDLS spectra of SiNPs (blue curve) and GP-Ce6-SiNPs (purple curve).cUV-Vis absorbance of Ce6 (blue curve), SiNPs (gray curve), and GP-Ce6-SiNPs (orange curve). The inset image shows the UV absorbance of GP, GP-SiNPs, and GP-SiNPs treated with phenol-sulfuric acid (GP-SiNPs + phenol-sulfuric).dPL spectra of SiNPs (blue curve), Ce6 (gray curve), GP (black curve), and GP-Ce6-SiNPs (orange curve) (λex= 405 nm).eZeta potential of SiNPs, GP, GP-SiNPs, Ce6, and GP-Ce6-SiNPs.f1O2generation abilities of H2O, PBS, free Ce6, and GP-Ce6-SiNPs determined by using SOSG. Error bars represent the standard deviation obtained from three independent measurements. Source data are provided as a Source Data file Figure 2a shows the transmission electron microscopy (TEM) image of GP-Ce6-SiNPs, which appear as spherical particles with excellent monodispersibility. The size distribution (Inset in Fig. 2a ), calculated by the measurement of 200 particles, shows that the average size of GP-Ce6-SiNPs is about 2.7 nm, slightly larger than that of unmodified SiNPs (2.3 nm) (see Supplementary Fig. 1 ). Dynamic light scattering (DLS) measurement of GP-Ce6-SiNPs is given in Fig. 2b , revealing that naked SiNPs exhibit a hydrodynamic diameter of ~3.0 nm, relatively smaller than ~5.6 nm of GP-Ce6-SiNPs. Fig. 2 Characterization of GP-Ce6-SiNPs. a TEM image and corresponding size distribution (inset) of GP-Ce6-SiNPs. Scale bar: 20 nm. b DLS spectra of SiNPs (blue curve) and GP-Ce6-SiNPs (purple curve). c UV-Vis absorbance of Ce6 (blue curve), SiNPs (gray curve), and GP-Ce6-SiNPs (orange curve). The inset image shows the UV absorbance of GP, GP-SiNPs, and GP-SiNPs treated with phenol-sulfuric acid (GP-SiNPs + phenol-sulfuric). d PL spectra of SiNPs (blue curve), Ce6 (gray curve), GP (black curve), and GP-Ce6-SiNPs (orange curve) ( λ ex = 405 nm). e Zeta potential of SiNPs, GP, GP-SiNPs, Ce6, and GP-Ce6-SiNPs. f 1 O 2 generation abilities of H 2 O, PBS, free Ce6, and GP-Ce6-SiNPs determined by using SOSG. Error bars represent the standard deviation obtained from three independent measurements. Source data are provided as a Source Data file Full size image The modification of GP and Ce6 is further confirmed by UV-vis absorbance -photoluminescence (PL) spectra, Zeta potential and Fourier-transform infrared (FTIR) spectra. As depicted in Fig. 2c , the absorption spectrum of GP-Ce6-SiNPs displays three characteristic absorption peaks at 320 nm (assigned to SiNPs), 405 nm, and 660 nm (assigned to Ce6). It is worth noting that a new distinct absorption peak at 490 nm would appear (Inset in Fig. 2c ) when GP-SiNPs are treated with phenol-sulfuric acid. Upon the phenol-sulfuric acid treatment, the linked GP is hydrolyzed into monosaccharide, which is then rapidly dehydrated to form furfural derivative [45] . The resultant furfural derivative can combine with phenol to form orange-yellow furfural resin, exhibiting a new absorption peak at 490 nm [45] , which also confirms the successful conjugation of GP molecules with SiNPs. The amounts of linked GP and loaded Ce6 onto SiNPs can be quantified based on the corresponding calibration absorption curves (Supplementary Fig. 2 ), respectively. In addition, the stability of GP-Ce6-SiNPs is validated in a series of solutions with different pH values (pH 5.5~7.5) and solutions containing various intracellular species (e.g., 150 mM KCl, 2 mM MgSO 4 , 10 mM NaHCO 3 , 2 mM CaCl 2 , 20 mM glucose, and 1 mM bovine serum albumin (BSA)), as revealed in Supplementary Figs. 3 and 4 . As for PL spectra in Fig. 2d , GP-Ce6-SiNPs display two characteristic emission peaks at 520  and 670 nm under the excitation of 405 nm, which are originated from SiNPs and Ce6, respectively [46] . With regard to Zeta potential in Fig. 2e , the negatively charged Ce6 molecules (−2.1 mV) can be electrostatically adsorbed on the surface of positively charged GP-SiNPs (0.4 mV). In FTIR spectra (Supplementary Fig. 5 ), the typical Si–O vibration at 1080 cm −1 is observed in both SiNPs and GP-Ce6-SiNPs, while the characteristic C–N vibration at 1640–1690 cm −1 is only shown in GP-Ce6-SiNPs possibly owing to the binding reaction between SiNPs and GP. To investigate PDT effects of GP-Ce6-SiNPs, singlet oxygen sensor green (SOSG) testing is employed. As shown in Fig. 2f , the 1 O 2 generation ability of GP-Ce6-SiNPs is similar to that of free Ce6 at the same Ce6 concentration under 660-nm irradiation, demonstrating distinct PDT ability of the GP-Ce6-SiNPs. In vitro imaging of diverse bacteria We first perform experiments to investigate whether GP-Ce6-SiNPs could target different kinds of bacteria in a specific manner. Gram-positive bacteria of S. aureus (SA), M. luteus (ML), and Gram-negative bacteria of E. coli (EC), P. aeruginosa (PA) are, respectively, incubated with GP-Ce6-SiNPs at 37 °C for 2 h, and then washed with phosphate buffered saline (PBS) buffer. As shown in the confocal laser scanning microscope (CLSM) images in Fig. 3a , both green fluorescence signals from the SiNPs (first column, λ ex = 405 nm, λ em = 500–550 nm) and red fluorescence signals from the Ce6 (second column, λ ex = 405 nm, λ em = 600–680 nm) can be clearly observed in all treated bacteria, indicating that GP-Ce6-SiNPs can specifically target Gram-positive and Gram-negative bacteria. Furthermore, green fluorescence signals overlap well with red fluorescence signals in the merged channel (third column) with Pearson correlation coefficients more than 0.80, demonstrating good colocalization between SiNPs and Ce6 ascribed to the good stability of GP-Ce6-SiNPs in the cellular environments. Also, there is no significant difference in intensity profiles of green and red signals within the ROI (region of interest, yellow lines in ML of Fig. 3a ) across bacteria cells (Fig. 3b ). To further test the role of GP in GP-Ce6-SiNPs for targeting bacteria, bacteria incubated with Ce6-modified SiNPs (Ce6-SiNPs) under the same conditions are selected for comparison. As shown in Supplementary Fig. 6 , no fluorescence signals are detected in bacteria treated with Ce6-SiNPs owing to the absence of GP molecules for targeting bacteria. On the other aspect, GP- and Ce6-modified silicon nanorods (GP-Ce6-SiNRs) are tested as another control group because they have the same surface modifications as GP-Ce6-SiNPs, but the size of GP-Ce6-SiNRs (~100 nm) is much larger than that of GP-Ce6-SiNPs (~2.7 nm) [47] . As revealed in Supplementary Fig. 7 , distinct fluorescence can not be observed in these four kinds of bacteria incubated with GP-Ce6-SiNRs, indicating larger-size nanoagents modified with GP ligand still can not be internalized into bacterial cells. Supplementary Fig. 8 shows systemic characterizations of Ce6-SiNPs and GP-Ce6-SiNRs, including TEM images, PL spectra, and UV-vis absorbance (see Supplementary Methods for details of the preparation of GP-Ce6-SiNRs). Fig. 3 In vitro imaging of Gram-negative and Gram-positive bacteria. a Confocal fluorescence images of four different kinds of bacteria (EC, SA, ML, and PA) after incubation with GP-Ce6-SiNPs. Scale bar: 10 μm. b Intensity profiles of ROI across the line shown in ML in panel ( a ) with confocal microscope. c Confocal fluorescence images of EC and SA treated with NaN 3 and then incubated with GP-Ce6-SiNPs for 2 h. Scale bar: 10 μm. d Confocal fluorescence images of EC and SA incubated with GP with different concentrations (0, 2, 20 mg mL −1 ) for 5 min and then incubated with GP-Ce6-SiNPs for 2 h. Scale bar: 25 μm. e TEM (scale bar: 1 μm) and zoom-in TEM (scale bar: 30 nm) images of intact EC and cell membrane of EC treated with GP-Ce6-SiNPs. f TEM (scale bar: 20 nm) and zoom-in TEM (scale bar: 5 nm) images of GP-Ce6-SiNPs nanoparticles in cell lysate of EC. g Confocal fluorescence images of the mixture of ARPE cells and EC, pure ARPE cells, the mixture of human blood and EC, pure human blood after incubation with GP-Ce6-SiNPs. Scale bar: 25 μm. h Histogram quantifying the level of GP-Ce6-SiNPs transport. Statistical analysis was performed using a one-way ANOVA analysis. Error bars represent the standard deviation obtained from three independent measurements (*** p < 0.001, n = 3). In the above experiments, the final concentration of GP-Ce6-SiNPs is 10 mg mL −1 (3.6 mg mL −1 of GP and 100 μg mL −1 of Ce6). Source data are provided as a Source Data file Full size image To examine if the uptake of GP-Ce6-SiNPs is mediated by energy-dependent transporter pathway, the accumulation of GP-Ce6-SiNPs within bacterial cells under 4 °C is observed by CLSM. As observed in Supplementary Fig. 9 , neither green nor red fluorescence signals could be clearly observed when the bacteria are incubated with GP-Ce6-SiNPs at 4 °C for 2 h. Such temperature-dependent internalization process indicates GP-Ce6-SiNPs transport into bacterial cells through energy-dependent transporter pathway. Furthermore, the inhibition assay as well as competition assay have been performed to confirm the uptake mechanism of GP-Ce6-SiNPs into bacteria via ABC transporter pathway. For the inhibition assay, sodium azide (NaN 3 ) is incubated with bacteria in order to inhibit the ATP-dependent ABC transporter pathway since NaN 3 can serve as the inhibitor of the respiratory chain of bacteria [48] . As a result, fluorescence is undetectable in the NaN 3 -treated EC and SA (Fig. 3c ) , indicating the accumulation of GP-Ce6-SiNPs into bacteria has been drastically inhibited. As for a competition assay, the EC and SA solutions are incubated with GP with concentrations of 0, 2, and 20 mg mL −1 for 5 min and then incubated with GP-Ce6-SiNPs for 2 h. Since GP molecules are internalized into bacterial cells also through ABC transporter pathway [36] , they would compete with GP-Ce6-SiNPs for ABC transporter. As a consequence, the fluorescence observed in bacteria becomes gradually weaken with the increase of GP concentrations (Fig. 3d ), suggesting the uptake of GP-Ce6-SiNPs into bacteria is greatly competitively inhibited by GP. On the other side, TEM characterizations of GP-Ce6-SiNPs stained EC are further performed to confirm whether GP-Ce6-SiNPs specifically enter into bacterial intracellular volume rather than nonspecifically adsorb on the bacteria cell surface. Typically, the surface of cell membrane of stained EC is smooth (see TEM images in Fig. 3e ), while numerous nanoparticles are observed in the lysate of stained EC cells (see TEM images in Fig. 3f ), demonstrating GP-Ce6-SiNPs are internalized into bacterial cells, but not binding to the bacteria cell surface. In order to investigate the specificity of GP-Ce6-SiNPs for bacteria over mammalian cells, HeLa cells, ARPE cells and human blood samples are selected for study. As revealed in confocal images in Fig. 3g , no fluorescence signals can be detected in pure ARPE cells, while green and red fluorescence signals are only observed in EC cells when ARPE cells are mixed with EC, followed by 2-h incubation with GP-Ce6-SiNPs. Moreover, green and red fluorescence signals are only observed in EC cells when human blood samples spiked with EC are treated with GP-Ce6-SiNPs for 2 h, suggesting the potential use of GP-Ce6-SiNPs for imaging of bacteria in clinical blood samples. 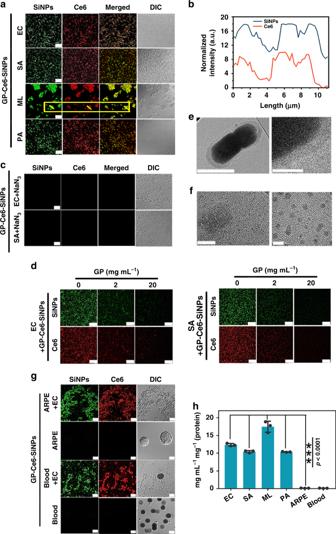Fig. 3 In vitro imaging of Gram-negative and Gram-positive bacteria.aConfocal fluorescence images of four different kinds of bacteria (EC, SA, ML, and PA) after incubation with GP-Ce6-SiNPs. Scale bar: 10 μm.bIntensity profiles of ROI across the line shown in ML in panel (a) with confocal microscope.cConfocal fluorescence images of EC and SA treated with NaN3and then incubated with GP-Ce6-SiNPs for 2 h. Scale bar: 10 μm.dConfocal fluorescence images of EC and SA incubated with GP with different concentrations (0, 2, 20 mg mL−1) for 5 min and then incubated with GP-Ce6-SiNPs for 2 h. Scale bar: 25 μm.eTEM (scale bar: 1 μm) and zoom-in TEM (scale bar: 30 nm) images of intact EC and cell membrane of EC treated with GP-Ce6-SiNPs.fTEM (scale bar: 20 nm) and zoom-in TEM (scale bar: 5 nm) images of GP-Ce6-SiNPs nanoparticles in cell lysate of EC.gConfocal fluorescence images of the mixture of ARPE cells and EC, pure ARPE cells, the mixture of human blood and EC, pure human blood after incubation with GP-Ce6-SiNPs. Scale bar: 25 μm.hHistogram quantifying the level of GP-Ce6-SiNPs transport. Statistical analysis was performed using a one-way ANOVA analysis. Error bars represent the standard deviation obtained from three independent measurements (***p< 0.001,n= 3). In the above experiments, the final concentration of GP-Ce6-SiNPs is 10 mg mL−1(3.6 mg mL−1of GP and 100 μg mL−1of Ce6). Source data are provided as a Source Data file Figure 3h shows higher level of GP-Ce6-SiNPs transporting in bacterial cells than in mammalian cells. Quantitatively, the amount of GP-Ce6-SiNPs accumulated into both Gram-positive and Gram-negative bacteria is at least 12 times more than that in ARPE and human blood cells. On the other aspect, the observed non-specific internalization of the nanoagents by mammalian cells might be mediated by the other pathway of endocytosis [49] . In vivo imaging of diverse bacteria To demonstrate that the as-prepared GP-Ce6-SiNPs have the potential to realize imaging of Gram-negative and Gram-positive bacteria in vivo, the corresponding bacteria-infected mice models are constructed. Micrograph of the histology of SA-infected muscles of mice in Fig. 4a shows that SA cells exist in infected tissues. In Fig. 4b and Fig. 4c , 50 μL SA with 0.9 × 10 7 CFU and 50 μL PA with 0.7 × 10 7 CFU are, respectively, injected into the right and left caudal thigh of mice. After 24-h infection, the treated mice are intravenously injected with 100 μL of vancomycin-modified SiNPs (Van-SiNPs) (Fig. 4b ) and GP-Ce6-SiNPs (Fig. 4c ) with the same amount of SiNPs (10 mg mL −1 ) through the tail vein, which are then imaged by an in vivo optical imaging system (IVIS Lumina III) under two channels of λ ex = 460 nm, λ em = 520 nm and λ ex = 460 nm, λ em = 670 nm at 24 h post injection. The actual amount of SA or PA at the infection site during imaging is 1.0 × 10 7 CFU, which is determined via tissue harvesting, homogenization, and culturing with CFU count [7] , [50] . As shown in Fig. 4b , Van-SiNPs can image SA infection while are unable to image PA infection, this result is consistent with the previous report, in which Van-SiNPs could only be specifically against Gram-positive bacteria based on the strong affinity between vancomycin and cell wall of Gram-positive bacteria [51] . As supported by corresponding histograms in Fig. 4b , in Van-SiNPs-treated mice, SA-infected site has a ~3.7-fold increase in fluorescence intensity compared with the PA - infected site. On the contrary, in GP-Ce6-SiNPs-treated groups, green and red fluorescence signals can be observed at both two infected sites (Fig. 4c ). And there is no significant difference of fluorescence intensity between the two sites, as reveled in corresponding histograms in Fig. 4c . In Fig. 4d , 50 μL PBS buffer and 50 μL the mixture containing PA and SA (PA + SA) with 0.8 × 10 7 CFU are, respectively, injected into the left and right caudal thigh of mice. After 24-h infection, the infected mice are intravenously injected with 100 μL of GP-Ce6-SiNPs and then imaged at 24 h post injection. The actual amount of mixed bacteria at the infection site during imaging is 1.0 × 10 7 CFU, which is determined by CFU counting method as mentioned above. Distinct green and red fluorescence signals can only be observed at the mixed bacteria-infected site instead of the PBS-treated site, as shown in Fig. 4d . In particular, the corresponding histograms in Fig. 4d show that the site of mice infected with PA + SA have a ~6.2-fold increase in fluorescence intensity compared with PBS-treated site. These experimental results indicate the GP-Ce6-SiNPs can achieve in vivo imaging of both Gram-negative and Gram-positive bacterial infections. Also, there exist negligible non-specific interactions between nanoparticles without GP (Ce6-SiNPs) and biological tissues, as demonstrated in Supplementary Fig. 10 . Fig. 4 In vivo imaging of infections caused by Gram-negative and Gram-positive bacteria. a Micrograph of the histology of 1.0 × 10 7 CFU of SA-infected and PBS-treated muscles. Scale bar: 50 μm. b In vivo imaging of 1.0 × 10 7 CFU of SA (right side) and 1.0 × 10 7 CFU of PA (left side)-infected sites of mice treated with Van-SiNPs and corresponding histograms of fluorescence intensity at two sites. c In vivo dual-emission imaging of 1.0 × 10 7 CFU of SA (right side) and 1.0 × 10 7 CFU of PA (left side)-infected sites of mice treated with GP-Ce6-SiNPs and corresponding histograms of fluorescence intensity at two sites. d In vivo dual-emission imaging of 1.0 × 10 7 CFU of mixture of PA and SA (PA + SA, right side) and PBS (left side)-treated sites of mice injected with GP-Ce6-SiNPs and corresponding histograms of fluorescence intensity at two sites. e In vivo dual-emission imaging of 1.0 × 10 5 CFU of SA or PA (right side) and PBS (left side)-treated sites of mice injected with GP-Ce6-SiNPs and corresponding histograms of fluorescence intensity at two sites. f Long-term in vivo dual-emission imaging of 1.0 × 10 7 CFU of SA-infected site of mice injected with GP-Ce6-SiNPs and corresponding time-dependent histograms of fluorescence intensity. The amount of bacteria at the infection site during imaging is determined via tissue harvesting, homogenization and culturing with CFU count. Statistical analysis was performed using paired two-tailed t -test. Error bars represent the standard deviation obtained from three independent measurements (*** p < 0.001, n = 3). The number ( n ) of mice in each experiment is 3, the total number is 18, and the gender of all mice is female. The cartoons are created by Dr. Houyu Wang. Source data are provided as a Source Data file Full size image The minimum number of bacteria imaged by GP-Ce6-SiNPs in vivo is determined in the following experiments. Fifty microliters of PBS buffer and 50 μL SA with 1.4 × 10 5 CFU or PA with 1.2 × 10 5 CFU are, respectively, injected into the left and right thigh of the mice and imaged by GP-Ce6-SiNPs. The actual amount of SA or PA at the infection site during imaging is determined as 1.0 × 10 5 CFU by using the same CFU counting method as mentioned above. 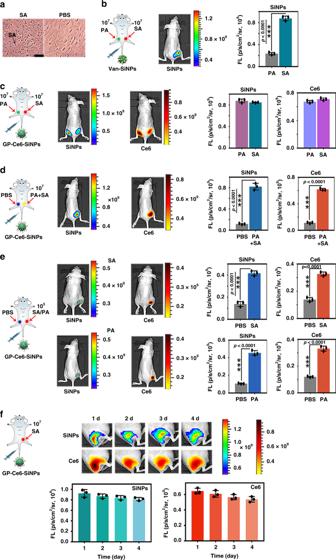Fig. 4 In vivo imaging of infections caused by Gram-negative and Gram-positive bacteria.aMicrograph of the histology of 1.0 × 107CFU of SA-infected and PBS-treated muscles. Scale bar: 50 μm.bIn vivo imaging of 1.0 × 107CFU of SA (right side) and 1.0 × 107CFU of PA (left side)-infected sites of mice treated with Van-SiNPs and corresponding histograms of fluorescence intensity at two sites.cIn vivo dual-emission imaging of 1.0 × 107CFU of SA (right side) and 1.0 × 107CFU of PA (left side)-infected sites of mice treated with GP-Ce6-SiNPs and corresponding histograms of fluorescence intensity at two sites.dIn vivo dual-emission imaging of 1.0 × 107CFU of mixture of PA and SA (PA + SA, right side) and PBS (left side)-treated sites of mice injected with GP-Ce6-SiNPs and corresponding histograms of fluorescence intensity at two sites.eIn vivo dual-emission imaging of 1.0 × 105CFU of SA or PA (right side) and PBS (left side)-treated sites of mice injected with GP-Ce6-SiNPs and corresponding histograms of fluorescence intensity at two sites.fLong-term in vivo dual-emission imaging of 1.0 × 107CFU of SA-infected site of mice injected with GP-Ce6-SiNPs and corresponding time-dependent histograms of fluorescence intensity. The amount of bacteria at the infection site during imaging is determined via tissue harvesting, homogenization and culturing with CFU count. Statistical analysis was performed using paired two-tailedt-test. Error bars represent the standard deviation obtained from three independent measurements (***p< 0.001,n= 3). The number (n) of mice in each experiment is 3, the total number is 18, and the gender of all mice is female. The cartoons are created by Dr. Houyu Wang. Source data are provided as a Source Data file Figure 4e presents that GP-Ce6-SiNPs can discriminate as few as 10 5 CFU of SA or PA in vivo under green and red emission channels. As revealed in corresponding histograms in Fig. 4e , the site of mice infected with 10 5 CFU of SA or PA have a ~2.7-fold or ~3.5-fold increase in fluorescence intensity compared with PBS-treated site. 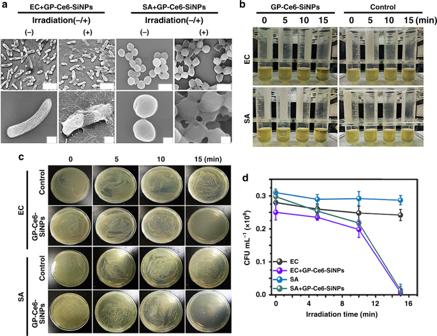Fig. 5 In vitro antibacterial activity of GP-Ce6-SiNPs.aSEM images of GP-Ce6-SiNPs-treated EC and SA before and after constant 660-nm irradiation (12 mW cm−2) for 15 min (scale bar in the first row: 1 μm, scale bar in the second row: 200 nm).bThe turbidity of EC and SA suspensions treated without GP-Ce6-SiNPs (control groups) or with GP-Ce6-SiNPs under constant irradiation (660 nm, 12 mW cm−2) for 0, 5, 10, and 15 min. The irradiation treatment on each sample is performed for one time.cPhotographs of the agar plates of EC and SA treated without (control groups) or with GP-Ce6-SiNPs under constant irradiation (660 nm, 12 mW cm−2) for 0, 5, 10, and 15 min.d, The corresponding bacterial counts (CFU mL−1) in panel (c). Error bars represent the standard deviation obtained from three independent measurements. The concentration of GP-Ce6-SiNPs is 10 mg mL−1(3.6 mg mL−1of GP and 100 μg mL−1of Ce6). Source data are provided as a Source Data file Furthermore, the developed GP-Ce6-SiNPs can be employed for long-term tracking bacterial infections in vivo by virtue of their good photostability and high specificity, as demonstrated in Fig. 4f . Typically, 50 μL SA (0.9 × 10 7 CFU) is injected into the right thigh muscle of mice. The mice are intravenously injected with 100 μL of GP-Ce6-SiNPs after 24-h infection. The actual amount of SA at the infection site during imaging is 1.0 × 10 7 CFU. As displayed in Fig. 4f , strong fluorescence signals from both SiNPs and Ce6 channels can still be observed at the infected site even at 4th day post injection. The corresponding time-dependent histograms in Fig. 4f show that fluorescence intensities from SiNPs and Ce6 keep steady at the infected site during 4-day treatment (e.g., the fluorescence intensity only drops by 12% at the 4th day compared with that at the 1st day), suggesting long retention ability of GP-Ce6-SiNPs at the infected site. In vitro antibacterial activity of GP-Ce6-SiNPs The in vitro antibacterial activity of GP-Ce6-SiNPs is evaluated by scanning electron microscope (SEM) characterizations, agar plate experiments, and liquid medium turbidity assays. In these antibacterial assays, EC and SA are chosen as the representative Gram-negative and Gram-positive bacteria. As shown in SEM images in Fig. 5a , smooth cell walls of EC and SA incubated with GP-Ce6-SiNPs for 2 h can be observed prior to light irradiation. On the contrary, rough and wrinkled cell walls and lysed debris of such EC and SA are found after treatment with light irradiation for 15 min (660 nm, 12 mW cm −2 ). As shown in Fig. 5b , luria-bertani (LB) liquid media in GP-Ce6-SiNPs-treated groups are pellucid due to the destruction of bacteria under constant 15-min irradiation, while the media become turbid in the control groups due to the rapid growth of bacteria. Nearly no bacterial colony of EC and SA exists in the group under constant 15-min irradiation. In contrast, numerous bacterial colonies are observed in control groups under the identical conditions (Fig. 5c ). For a more reliable quantitative measurement, irradiation time-dependent CFU counting is performed, as shown in Fig. 5d . The bacterial counts of groups of EC and SA treated with GP-Ce6-SiNPs under constant 15-min irradiation drop dramatically compared to control groups under the same conditions. These experimental results demonstrate the in vitro photodynamic antimicrobial activity of GP-Ce6-SiNPs. Fig. 5 In vitro antibacterial activity of GP-Ce6-SiNPs. a SEM images of GP-Ce6-SiNPs-treated EC and SA before and after constant 660-nm irradiation (12 mW cm −2 ) for 15 min (scale bar in the first row: 1 μm, scale bar in the second row: 200 nm). b The turbidity of EC and SA suspensions treated without GP-Ce6-SiNPs (control groups) or with GP-Ce6-SiNPs under constant irradiation (660 nm, 12 mW cm −2 ) for 0, 5, 10, and 15 min. The irradiation treatment on each sample is performed for one time. c Photographs of the agar plates of EC and SA treated without (control groups) or with GP-Ce6-SiNPs under constant irradiation (660 nm, 12 mW cm −2 ) for 0, 5, 10, and 15 min. d , The corresponding bacterial counts (CFU mL −1 ) in panel ( c ). 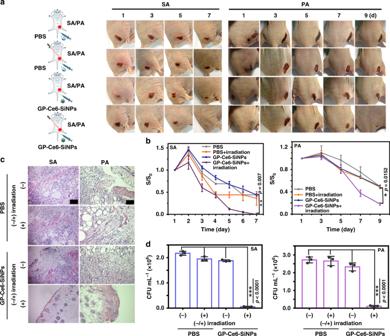Fig. 6 In vivo antibacterial activity of GP-Ce6-SiNPs.aRepresentative photographs of time-dependent of SA- and PA-infected mice injected with GP-Ce6-SiNPs or PBS treated with or without light irradiation (660 nm, 12 mW cm−2) for constant 40 min. The cartoons are created by Dr. Houyu Wang.bCorresponding time-dependent relative wound area (S/S0) of SA- and PA-infected mice in panel (a). S0stands for the size of infection site at 1-day treatment and S stands for the size of infection site atn-day treatment. Error bars represent the standard deviation obtained from three independent measurements.cCorresponding histological images of the SA- and PA-infected skin tissues of mice in panel (a) at the 7th (SA) and 9th day (PA) post injection. Scale bar: 100 μm.dBacterial counts (CFU mL−1) excised from the SA- and PA-infected tissues of mice at the 7th (SA) and 9th (PA) day post injection. Statistical analysis was performed using a one-way ANOVA analysis. Error bars represent the standard deviation obtained from three independent measurements (*p< 0.05, **p< 0.01, ***p< 0.001,n= 3). The concentration of GP-Ce6-SiNPs is 10 mg mL−1(3.6 mg mL−1of GP and 100 μg mL−1of Ce6). Typically, the number (n) of mice used per experiment is 3, the total number is 24, and the gender of mice is female. Source data are provided as a Source Data file 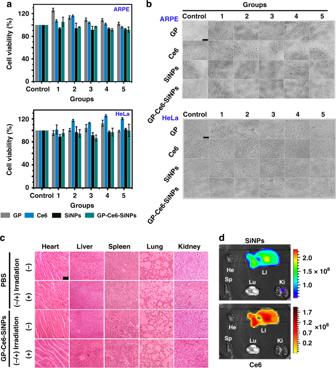Fig. 7 In vitro and in vivo toxicity tests. Cell viability (a) and morphology (b) of ARPE (up, normal cells) and HeLa cells (down, cancer cells) treated with different dosages of GP, Ce6, SiNPs, and GP-Ce6-SiNPs for 24 h, respectively. The groups of “Control, 1, 2, 3, 4, 5” represent series of concentrations of GP (0, 5, 2.5, 1.25, 0.625, 0.313 mg mL−1), Ce6 (0, 100, 50, 25, 12.5, 6.25 μg mL−1), SiNPs and GP-Ce6-SiNPs (0, 10, 5, 2.5, 1.25, 0.625 mg mL−1). All error bars represent the standard deviation determined from three independent assays. Scale bar: 50 μm.cHistological evaluation of different organs (heart, liver, spleen, lung, and kidney) from healthy mice, which are suffered from 10-day treatment of PBS, PBS + irradiation, GP-Ce6-SiNPs, GP-Ce6-SiNPs + irradiation, respectively. Scale bar: 100 μm.dEx vivo dual-emission imaging of organs resected from healthy mice after 24 h post injection of GP-Ce6-SiNPs. First row (from left to right): heart (He), liver (Li); second row (from left to right): spleen (Sp), lung (Lu), and kidney (Ki). Source data are provided as a Source Data file Error bars represent the standard deviation obtained from three independent measurements. The concentration of GP-Ce6-SiNPs is 10 mg mL −1 (3.6 mg mL −1 of GP and 100 μg mL −1 of Ce6). Source data are provided as a Source Data file Full size image In vivo antibacterial activity of GP-Ce6-SiNPs To further evaluate the antibacterial ability of GP-Ce6-SiNPs in vivo, 50 μL of SA (1.0 × 10 7 CFU) and PA (1.0 × 10 7 CFU) are injected into the right thigh of the mice, respectively. Then these two groups of bacteria (SA, PA)-infected mice are intravenously injected with 100 μL of PBS and GP-Ce6-SiNPs under 660-nm irradiation, respectively; the other two groups of infected mice are suffered from the same treatments but without 660-nm irradiation. The representative photographs of four groups of bacteria (SA, PA)-infected mice are shown in Fig. 6a . Typically, among these four groups, the earliest and fastest infection wound healing and scarring is observed in the mice treated with GP-Ce6-SiNPs coupled with irradiation at 660 nm (12 mW cm −2 ) for 40 min. Moreover, the corresponding infection wound area is measured every day and the relative wound area (S/S 0 ) is plotted in Fig. 6b . The comparisons of the relative wound area among the experimental groups and control groups have been made for both SA- and PA-infected mice. Particularly, in SA-infected mice, a significant difference ( p < 0.01) exists among the nanoagent + irradiation, the PBS and nanoagent alone. On the contrary, no significant difference exists between the nanoagent + irradiation and PBS + irradiation, which might be due to the adaptable self-healing ability of mice toward SA infections. On the other aspect, for PA-infected mice, a significance comparison ( p < 0.05) in the relative wound area is made among the nanoagent + irradiation, the PBS + irradiation, the PBS and nanoagent alone. The corresponding hematoxylin-eosin (H&E) staining images of infection tissues of four groups from SA- and PA-infected mice at 7th (SA) and 9th (PA) day treatment are exhibited in Fig. 6c . Normal morphological features with blood vessels and hair follicles can be detected in all groups treated with GP-Ce6-SiNPs under light irradiation while the tissues from other three control groups are damaged, emerging a large number of neutrophils. Additionally, the SA- and PA-infected skin tissues are excised from the mice at the 7th (SA) and 9th (PA) day post injection and the amounts of bacteria collected from the excised tissues are measured to assess antibacterial rates. As depicted in Fig. 6d , the amounts of bacteria in the “nanoagent + irradiation” groups are significantly ( p < 0.001) less than the other control groups. Quantitatively, the antibacterial rate of GP-Ce6-SiNPs is calculated as 98% against SA and 96% against PA. These experimental results suggest significant photodynamic antimicrobial activity of GP-Ce6-SiNPs in vivo. Fig. 6 In vivo antibacterial activity of GP-Ce6-SiNPs. a Representative photographs of time-dependent of SA- and PA-infected mice injected with GP-Ce6-SiNPs or PBS treated with or without light irradiation (660 nm, 12 mW cm −2 ) for constant 40 min. The cartoons are created by Dr. Houyu Wang. b Corresponding time-dependent relative wound area (S/S 0 ) of SA- and PA-infected mice in panel ( a ). S 0 stands for the size of infection site at 1-day treatment and S stands for the size of infection site at n -day treatment. Error bars represent the standard deviation obtained from three independent measurements. c Corresponding histological images of the SA- and PA-infected skin tissues of mice in panel ( a ) at the 7th (SA) and 9th day (PA) post injection. Scale bar: 100 μm. d Bacterial counts (CFU mL −1 ) excised from the SA- and PA-infected tissues of mice at the 7th (SA) and 9th (PA) day post injection. Statistical analysis was performed using a one-way ANOVA analysis. Error bars represent the standard deviation obtained from three independent measurements (* p < 0.05, ** p < 0.01, *** p < 0.001, n = 3). The concentration of GP-Ce6-SiNPs is 10 mg mL −1 (3.6 mg mL −1 of GP and 100 μg mL −1 of Ce6). Typically, the number ( n ) of mice used per experiment is 3, the total number is 24, and the gender of mice is female. Source data are provided as a Source Data file Full size image Toxicity assessment of GP-Ce6-SiNPs Cytotoxicity of GP-Ce6-SiNPs is evaluated by an established methyl thiazolyl tetrazolium (MTT) assays. As shown in Fig. 7a , the cell viability of HeLa and ARPE cells remains above 90% when they are incubated with GP-Ce6-SiNPs with different concentrations for 24 h. The corresponding images of morphologies of treated cells are presented in Fig. 7b , showing there is no obvious morphological change in HeLa or ARPE cells incubated with GP-Ce6-SiNPs. These results suggest feeble cytotoxicity of GP-Ce6-SiNPs. Afterward, in vivo biocompatibility of GP-Ce6-SiNPs is investigated. The main organs of heart, liver, spleen, lung, and kidney are resected from PBS/nanoagents-treated healthy mice with or without irradiation after 10-day treatment. As revealed in Fig. 7c , normal morphological features are found in biopsy sections in all resected organs, implying the negligible toxicity of GP-Ce6-SiNPs in vivo. To further evaluate the biodistribution of GP-Ce6-SiNPs, ex vivo imaging of heart, liver, spleen, lung, and kidney resected from healthy mice after 24 h post injection of GP-Ce6-SiNPs is performed. As indicated in Fig. 7d , bright green and red fluorescence signals are only observed in liver and kidney rather than in other organs, indicating GP-Ce6-SiNPs are mainly metabolized by liver and not retained in other organs. Moreover, ex vivo imaging of the urine collected from the healthy mice after 4 h post injection of nanoagents is performed. As shown in Supplementary Fig. 11 , green and red fluorescence signals are observed in urine from the mice treated with nanoagents, confirming that nanoagents can be eliminated from the mice through renal clearance owing to the small size of nanoagents (~2.7 nm), which is in a good agreement with previous reports [52] , [53] These results demonstrate negligible in vitro and in vivo toxicity of GP-Ce6-SiNPs. Besides, the irradiation of PDT produces feeble toxicity in mammalian cells in vivo (Supplementary Fig. 12 ). Fig. 7 In vitro and in vivo toxicity tests. Cell viability ( a ) and morphology ( b ) of ARPE (up, normal cells) and HeLa cells (down, cancer cells) treated with different dosages of GP, Ce6, SiNPs, and GP-Ce6-SiNPs for 24 h, respectively. The groups of “Control, 1, 2, 3, 4, 5” represent series of concentrations of GP (0, 5, 2.5, 1.25, 0.625, 0.313 mg mL −1 ), Ce6 (0, 100, 50, 25, 12.5, 6.25 μg mL −1 ), SiNPs and GP-Ce6-SiNPs (0, 10, 5, 2.5, 1.25, 0.625 mg mL −1 ). All error bars represent the standard deviation determined from three independent assays. Scale bar: 50 μm. c Histological evaluation of different organs (heart, liver, spleen, lung, and kidney) from healthy mice, which are suffered from 10-day treatment of PBS, PBS + irradiation, GP-Ce6-SiNPs, GP-Ce6-SiNPs + irradiation, respectively. Scale bar: 100 μm. d Ex vivo dual-emission imaging of organs resected from healthy mice after 24 h post injection of GP-Ce6-SiNPs. First row (from left to right): heart (He), liver (Li); second row (from left to right): spleen (Sp), lung (Lu), and kidney (Ki). Source data are provided as a Source Data file Full size image The presented multifunctional nanoagents are made of SiNPs functionalized with GP and loaded with Ce6. In the as-prepared nanoagents, GP, serving as ideal targeted ligand for imaging bacteria, is covalently linked to SiNPs. Of note, the structural modifications at the reducing end of GP would not influence the internalization of probes by ABC transporters because the nonreducing end of GP was hypothesized as the recognized site of ABC transporters [36] , [37] . Another noticeable feature of nanoagents is that the green fluorescent emission from SiNPs under 405-nm UV excitation is not desirable for in vivo imaging due to its relatively poor penetration depth. To circumvent this issue, Ce6 loaded on SiNPs serves not only as a PDT agent but also as an imaging agent to provide stable red fluorescence signal (maximum emission wavelength at 670 nm), facilitating the improvement of the penetration depth. Notwithstanding, it is also important to develop near-infrared light-emitting SiNPs-based probes in the future, facilitating the improvement of the penetration depth of tissues in vivo. There are two prerequisites for nanoagents to access bacterial cells through the ABC transporter pathway: (1) surface modification of nanoagents with glucosyl residues and (2) relative small size of nanoagents. In this case, the as-prepared GP-Ce6-SiNPs can be selectively internalized into both Gram-negative and Gram-positive bacterial cells, while hardly entering mammalian cells. The high specificity of GP-Ce6-SiNPs for bacteria over mammalian cells is mainly ascribed to two factors: (1) GP-mediated ABC transporters are only presented in bacteria rather than in mammalian cells, and thus mammalian cells can not internalize SiNPs conjugated to GP ligand; (2) GP is composed of hydrophilic α (1–4)-linked glucose oligomer, which is unable to penetrate mammalian cellular membrane, resulting in low levels of non-specific uptake in mammalian cells [36] , [54] . Occasionally, the nanoagents might be nonspecifically internalized into mammalian cells by the pathway of endocytosis. However, the uptake rate mediated by endocytosis is much lower than that mediated by ABC-transporter pathway. Importantly, the minimum number of bacteria discriminated in vivo by nanoagents is 10 5 CFU. Bacteria at a concentration <10 5 CFU are hardly discriminated, which is probably due to the fact that 10 5 CFU of bacteria are too few to establish a stable infection in immune competent mice. Normally, the amount of bacteria would fluctuate in the intervening time between infection and imaging since the bacteria reproduce and are fought by the immune system. A reliable way to determine the amount of bacteria at the infection site during imaging in this study is tissue harvesting, homogenization and culturing with CFU count [7] , [50] . Moreover, the nanoagents can afford a long-term imaging (4 days) of bacterial infections in vivo, exhibiting stable green and red fluorescence signals. Finally, the antibacterial efficiency is up to ca. 98% against SA and ca. 96% against PA under 660-nm irradiation for constant 40 min with a relative low power density of 12 mW cm −2 . Such significant therapeutic effect is also attributed to selective and robust internalization of GP-Ce6-SiNPs into bacteria, resulting in a relative high local concentration of Ce6 at infection sites. The mechanism of the nanoagents against bacteria is based on photodynamic effect of Ce6, which is different from that of conventional antibiotics. It is worth noting that nanoagents amount used in our case is relatively high (10 mg mL −1 ), which is based on the following two considerations: (1) providing strong fluorescence signals even at ultralow concentrations of bacteria (e.g., 1.0 × 10 5 CFU mL −1 ); (2) achieving desirable treatment effects within a relatively short irradiation time to eliminate possible skin damage. Based on further optimizing experimental parameters (e.g., nanoagents amount) and systematical biosafety assessment, we envision that the developed multifunctional nanoagents with appropriate injection dose would hold potential applications for diagnosis and therapy of bacterial infections. Chemicals and reagents (3-aminopropyl) trimethoxysilane (C 6 H 17 NO 3 Si), 1,8-naphthalimide, vancomycin (Van), N-(3-dimethy-laminopropyl)-N′-ethylcarbodiimide-hydrochloride (EDC), N-hydroxysulfosuccinimide (NHS), trisodium citrate, citric acid and NaBH 4 were purchased from Sigma-Aldrich. E. coli (EC) (ATCC 11303), HeLa, and ARPE-19 cells were purchased from American Type Culture Collection (ATCC). S. aureus (SA) was obtained from the First Affiliated Hospital of Soochow University. M. luteus (ML) (BNCC 102589) and P. aeruginosa (PA) (BNCC 125486) were purchased from BeNa Culture Collection (BNCC). The human blood samples were provided by a healthy volunteer. All bacterial culture reagents (LB medium) were obtained from Sangon Biotech (Shanghai, China), and reagents for cellular culture were provided by Gibco (GrandIsland, USA). HeLa and ARPE-19 cells were cultured in Dulbecco’s modified Eagle’s medium (DMEM) and Roswell Park Memorial Institute (RPMI)-1640 medium, respectively. Both media were supplemented with 10% heat-inactivated fetal bovine serum (FBS) and relevant antibiotics (100 μg mL −1 streptomycin and 100 U mL −1 penicillin). Both cell lines were cultured at 37 °C in a 5% CO 2 incubator with humidified atmosphere. Six-week-old female nude mice (18–25 g in weight) were provided by Suzhou Pengsheng Biological Company. Propidium Iodide (PI), SYTO9, chlorin e6 (Ce6), and glucose polymer (GP) of poly[4-O-(α-D-glucopyranosyl)-D-glucopyranose] were purchased from Sigma-Aldrich (Shanghai, China). All animal experimental procedures were performed according to the Guideline for Animal Experimentation with the approval of the animal care committee of Soochow University. Instruments The morphology and size of nanoprobes were examined by transmission electronic microscopy (TEM, Philips CM 200) with 200 kV. A 750 UV-vis near-infrared spectrophotometer (Perkin-Elmer lambda) was used for the measurement of UV-vis absorption spectra. A spectro-fluorimeter (HORIBA JOBIN YVON FLUORMAX-4) was employed for recording photoluminescence (PL). FTIR spectrometer (Bruker HYPERION) was used for the characterization of FTIR spectra. Delsa™ nano submicron particle size and Zeta potential particle analyzer (Beckman Coulter, Inc) was employed for the analysis of dynamic light scattering (DLS) and Zeta potentials. Fluorescence imaging experiments were performed by a confocal laser scanning microscope (CLSM, Leica, TCS-SP5 II). In vivo fluorescence images were obtained by an in vivo optical imaging system (IVIS Lumina III). The number of bacterial colonies were counted by a colony counting instrument (Czone 8). Fabrication of GP-Ce6-SiNPs The SiNPs were synthesized in the presence of C 6 H 17 NO 3 Si and 1,8-naphthalimide molecules under 40 min of continuous UV irradiation at 365 nm at room temperature. To remove residual reactants, the resultant solution was purified by centrifugation at 6000 rpm for 15 min and dialysis (MWCO, 1000, Spectra/Pro). The final SiNPs solution was collected through evaporation and stored at 4 °C for future use. Next, the SiNPs solution (150 μL, 25 mg mL −1 ) was mixed with GP dissolved in deionized water (100 μL, 10 mg mL −1 ). The dispersion was continuously stirred at 70 °C for 6 h, and 0.01 mg of NaBH 4 was added and reacted for another 12 h at room temperature to obtain the stable GP-modified SiNPs. To remove the unreacted GP, the reaction solution was filtered by using Nanosep centrifugal devices (MW cutoff, 3 kDa; Millipore) through centrifugation at 7500 rpm for 15 min. To further fabricate the GP-Ce6-SiNPs, the Ce6 solution (50 μL, 200 μM) was added in the above prepared GP-SiNPs solution and stirred at room temperature overnight. Of note, excess free or unreacted Ce6 was removed using Nanosep centrifugal devices (MW cutoff, 3 kDa; Millipore) through centrifugation at 7000 rpm for 10 min. Then the product was collected and stored at 4 °C in the dark for the following experiments. Preparation of Van-SiNPs Hundred microliters of EDC (50 mg mL −1 ) and 25 µL of NHS (50 mg mL −1 ) was mixed with 5 mg Van powder at 4 °C under stirring for 15 min in order. Then, 50 µL of SiNPs solution (25 mg mL −1 ) was added into the activated Van solution for another 12 h at 4 °C in dark to obtain Van-SiNPs. To remove the excess unreacted Van, the resulting mixture was filtered by using Nanosep centrifugal devices (MW cutoff, 10 kDa; Millipore) through centrifugation at 7500 rpm for 15 min. The final mixture was stored at 4 °C in the dark. Bacterial culture Gram-negative EC and PA, Gram-positive SA and ML, were employed in experiments. Bacterial cells were grown in LB medium at 250 rpm and 37 °C and then obtained at the exponential growth phase. Finally, the bacterial suspensions were washed twice and re-suspended in PBS buffer for the next use. The concentration of bacteria was detected by measuring the optical density (OD) at 600 nm. Fluorescence imaging of bacteria and cells in vitro The 20 µL of purified and re-suspended bacterial suspension (1.0 × 10 7 CFU) was incubated with GP-Ce6-SiNPs (200 µL, 10 mg mL −1 ) for 2 h in a shaking incubator (200 rpm) at 37 °C. The bacteria were harvested by centrifuging the mixture at 8000 rpm for 10 min in Eppendorf (EP) tubes. The resulting bacteria were re-suspended and washed with PBS for three times. Then 10 µL of the washed bacteria solution was transferred onto a microscope slide covered by a coverslip, and then imaged by a confocal laser microscope with 30% power of diode laser. For the fluorescence imaging of mixture sample of bacteria and cells, ARPE cells were cultured in Dulbecco’s modified Eagle’s medium (DMEM) in 6-well cell culture plate at a density of 2.0 × 10 5 /well for 24 h (37 °C, 5% CO 2 ) and then mixed with EC bacterial suspension. The mixture of EC and ARPE cells were harvested by centrifuging the solutions at 8000 rpm for 10 min in EP tubes. The 20 µL of purified and re-suspended mixture suspension was incubated with GP-Ce6-SiNPs (200 µL, 10 mg mL −1 ) for 2 h in a shaking incubator (200 rpm) at 37 °C. Then 10 µL of the washed mixture solution was transferred onto a microscope slide covered by a coverslip, and imaged by a confocal laser microscope. Fluorescence imaging of the mixture of EC and human blood was obtained according to the same protocol above. Of note, the studies in human blood were conducted under a protocol that was reviewed and approved by the ethics committee. All fluorescence images were captured by CLSM (Leica, TCS-SP5 II) with a × 64 oil-immersion objective and taken under exactly the same optical conditions, and the same brightness and contrast was applied to the images by the microscope automatically. The processing and analysis of ROI was performed by the commercial image analysis software (Leica Application Suite Advanced Fluorescence Lite (LAS AF Lite)). Quantifying transport of nanoagents into bacteria The bacteria were incubated with nanoagents (200 µL, 10 mg mL −1 ) for 2 h, and then collected by centrifugation at 8000 rpm for 10 min. The collected bacteria solution was placed on an ice bath and lysed by sonication for 10 min, and the bacterial supernatant was isolated via centrifugation at 10,000 rpm for 10 min. Afterward, UV absorbance of nanoagents in the supernatant was measured to determine the concentration of nanoagents ( C nanoagent ) based on the calibration curve. On the other aspect, the bacterial protein mass ( M protein ) was quantified by the bicinchoninic acid (BCA) assay. As a consequence, the Y axis in Fig. 3h was generated, which was a normalized value of nanoagents content in bacterial supernatant ( C nanoagent / M protein ). In vivo imaging of bacterial infections To construct the bacteria-infected mice model, 50 μL of PA (0.7 × 10 7 CFU) and SA (0.9 × 10 7 CFU) were subcutaneously injected into the left and right caudal thigh of the mice. The actual amount of bacteria at the infection sites during imaging was determined via tissue harvesting, homogenization and culturing with CFU count. Specifically, the harvested tissues were first homogenized in sterile PBS buffer (1 mL). Then, the bacteria suspension was collected from the tissue dispersions by centrifugation (1000 rpm) removing tissue fragments. Finally, the collected bacteria were diluted by PBS buffer and cultured on an agarose medium at 37 °C for 12 h, followed by counting bacterial colonies by using a colony counting instrument (Czone 8). By using this method, the actual amount of SA or PA at the infection site during imaging is determined as 1.0 × 10 7 CFU. On the other aspect, 50 μL of PBS and 50 μL of mixture bacterial solution (PA + SA, 0.8 × 10 7 CFU) were subcutaneously injected into the left and right caudal thigh of the mice; the actual amount of mixed bacteria at the infection site during imaging is 1.0 × 10 7 CFU, which is determined by CFU counting method as mentioned above. Fifty microliters of PBS and 50 μL of SA (1.4 × 10 5 CFU) or PA (1.2 × 10 5 CFU) were subcutaneously injected into the left and right caudal thigh of the mice. The actual amount of SA or PA at the infection site during imaging is determined as 1.0 × 10 5 CFU by using the same CFU counting method as mentioned above. After 24 h post infection, bacteria-infected mice were intravenously injected with 100 μL GP-Ce6-SiNPs (10 mg mL −1 ) or 100 μL Van-SiNPs (10 mg mL −1 ) and then imaged by an in vivo optical imaging system (IVIS Lumina III) equipped with two laser channels of λ ex = 460 nm, λ em = 520 nm and λ ex = 460 nm, λ em = 670 nm at 24 h post injection. Meanwhile, the infected tissues cutoff from the mice were fixed in 4% paraformaldehyde (PFA) solution, mounted with paraffin, sliced, stained with Gram Stain Kits to detect the presence of bacteria. Of note, all studies in mice were conducted under a protocol that was reviewed and approved by the ethics committee. In vitro antibacterial assays The morphology of bacteria treated with GP-Ce6-SiNPs nanoagents (200 µL, 10 mg mL −1 ) before and after 660 nm light irradiation was characterized by SEM (FEI Quanta 200F). Bacterial suspensions treated with GP-Ce6-SiNPs before and after 660 nm light irradiation for 15 min were dropped onto silicon wafers, fixed by 4% PFA for 20 min at room temperature, and then dehydrated by ethanol with serial concentrations (e.g., 50, 75, 90, and 100% ethanol solutions, each for 5 min). Finally, the silicon wafers were completely dried and coated with gold for SEM measuring. As for the agar plates and turbidity assay, all samples were, respectively, constantly irradiated for 0, 5, 10, and 15 min at 660-nm irradiation. The irradiation treatment on each sample was performed for one time. The measurement was immediately performed after irradiation. In vivo antibacterial assays To evaluate photodynamic efficacy of GP-Ce6-SiNPs in vivo, the SA-infected or PA-infected mice were intravenously injected with 100 μL PBS and GP-Ce6-SiNPs (10 mg mL −1 ), respectively, and then divided into four groups including the group of PBS, PBS + light irradiation, GP-Ce6-SiNPs and GP-Ce6-SiNPs + light irradiation. The wound area was photographed and the size of wound area was processed by Image J software. At the last day of treatment, the bacteria extracted from the infected tissues of the mice ( n = 3) were cultured on the agar plates and the final bacteria colonies were counted to obtain the antibacterial rate. The percentage of antibacterial rate was generated on the basis of CFU counts from Fig. 6d . The antibacterial rate was calculated based on Eq. ( 1 ): 
    Antibacterial rate ( %) = ( N_control - N_experiment)/N_control× 100%
 (1) where N control and N experiment , respectively, stand for bacterial counts (CFU mL −1 ) from the groups of PBS (control) and GP-Ce6-SiNPs + irradiation (experiment) in Fig. 6d . The CFU counts in Fig. 6d were obtained from three independent measurements. For instance, N control and N experiment in S. aureus (SA)-infected tissues are 2.17 × 10 6 CFU mL −1 and 0.05 × 10 6 CFU mL −1 , and antibacterial rate is calculated as 98%; N control and N experiment in P. aeruginosa (PA)-infected tissues are 2.72 × 10 6 CFU mL −1 and 0.12 × 10 6 CFU mL −1 , and antibacterial rate is calculated as 96%. Meanwhile, the infected tissues from each group of mice were fixed in the 4% PFA solution for the following H&E staining. The photodynamic device in this research is a 660-nm light-emitting diode laser system with the beam diameter of 11 cm, so the infected area with the size of ~15 mm 2 was not scanned or rotated because the beam diameter of ~11 cm is large enough to cover whole mice body and also the infection site. The constant and static irradiation (660 nm, 12 mW cm −2 ) was employed on the bacteria samples and the mice According to “Laser Safety in the Health Care Environment (ANSI Z 136.1)” made by the American National Standards Institute (ANSI) (Laser Institute of American, 2014), the maximum permissible exposure (MPE) for skin exposure to a laser for wavelength from 400 to 700 nm is 0.2C A W cm −2 (C A = 1.0 under the 400–700 nm wavelength) when exposure duration is <3 × 10 4 s. We therefore confirm that the 12 mW cm −2 falls within the MPE guidelines and complies with the laser safety standard. In vitro and in vivo toxicity assessment The cytotoxicity assay was performed by using the cancer cells (HeLa) and the normal cells (ARPE) based on an established colorimetric MTT assay. Briefly, these cells were seeded into the 96-well cell culture plate at a density of 1.0 × 10 4 /well for 24 h (37 °C, 5% CO 2 ) and treated with serial concentrations of SiNPs (0, 10, 5, 2.5, 1.25, 0.625 mg mL −1 ), GP (0, 5, 2.5, 1.25, 0.625, 0.313 mg mL −1 ), Ce6 (0, 100, 50, 25, 12.5, 6.25 μg mL −1 ) and entire GP-Ce6-SiNPs (0, 10, 5, 2.5, 1.25, 0.625 mg mL −1 ), respectively. For each well, 20 μL stock MTT (5 mg mL −1 ) was added with further incubation at 37 °C for 6 h, and acidified sodium dodecyl sulfate (SDS) (100 μL/well) was used to lyse the cells. Finally, the cell viability was determined by measuring the absorbance at 570 nm with microplate reader (Bio-Rad 680, USA). All above experiments were performed for three independent measurements. For the biocompatibility evaluation of GP-Ce6-SiNPs in vivo, the main organs from PBS/nanoagents (100 µL, 10 mg mL −1 )-treated healthy mice with or without irradiation after 10-day treatment including the heart, liver, spleen, lung, and kidney were collected, fixed by 4% PFA solution, mounted with paraffin, sliced, stained with hematoxylin and eosin, and then imaged by a microscope. To investigate the biodistribution of GP-Ce6-SiNPs, ex vivo fluorescence imaging was carried out. The nanoagents (100 µL, 10 mg mL −1 )-treated healthy mice were sacrificed after 24 h post injection to collect the main organs for in vivo optical imaging. The urine of nanoagents (100 µL, 10 mg mL −1 )-treated healthy mice was collected after 4 h post injection and imaged by an in vivo optical imaging system. Statistical analysis Error bars represent the standard deviation obtained from three independent measurements. All the statistical analyses were performed using Origin software and GraphPad Prism software. The images were processed by Image J software. The statistical significance of differences was determined by a one-way ANOVA analysis or paired two-tailed t -test. p < 0.05 (*), p < 0.01 (**), and p < 0.001 (***) were used to indicate statistical difference. Reporting summary Further information on research design is available in the Nature Research Reporting Summary linked to this article.